Performance enhancement of metal nanowire transparent conducting electrodes by mesoscale metal wires For transparent conducting electrodes in optoelectronic devices, electrical sheet resistance and optical transmittance are two of the main criteria. Recently, metal nanowires have been demonstrated to be a promising type of transparent conducting electrode because of low sheet resistance and high transmittance. Here we incorporate a mesoscale metal wire (1–5 μm in diameter) into metal nanowire transparent conducting electrodes and demonstrate at least a one order of magnitude reduction in sheet resistance at a given transmittance. We realize experimentally a hybrid of mesoscale and nanoscale metal nanowires with high performance, including a sheet resistance of 0.36 Ω sq −1 and transmittance of 92%. In addition, the mesoscale metal wires are applied to a wide range of transparent conducting electrodes including conducting polymers and oxides with improvement up to several orders of magnitude. The metal mesowires can be synthesized by electrospinning methods and their general applicability opens up opportunities for many transparent conducting electrode applications. Transparent conducting electrodes (TCEs) are essential components for numerous optoelectronic devices that require transport of both electrons and photons, including solar cells, displays, touch screens and smart windows [1] , [2] , [3] , [4] , [5] . Recently, there have been increasing efforts in developing nanomaterial TCEs including carbon nanotubes (CNTs) [1] , [6] , [7] , [8] , [9] , graphene [4] , [10] , [11] , [12] , [13] , metal nanowires [14] , [15] , [16] , [17] , [18] , [19] , [20] , [21] and nanoparticles [22] , [23] to replace conventional indium tin oxide (ITO) films, in order to enable low-cost and mechanical flexibility while maintaining low sheet resistance ( R s ) and high transmittance ( T ). For the active layers of many devices, the lateral surface electrical conductance is sufficient to transport electrons only locally from several 100 nm to a few μm scale without serious ohmic loss, therefore interfacing with external connection requires additional TCEs with good R s –T performance. Based on the electrode structure, there are two types of TCEs: Type I is based on continuous films such as ITO, aluminum-doped zinc oxide (AZO), novel oxide, metal thin films, large-area graphene and conducting polymers. At T =90%, R s values for good ITO are 5–20 Ω sq −1 , for graphene 30–1,000 Ω sq −1 and for conducting polymers 100–450 Ω sq −1 , respectively [4] , [10] , [24] , [25] , [26] , [27] , [28] , [29] , [30] . Type II is based on networks of one-dimensional (1D) nanomaterials including CNTs, graphene nanoribbons, metal nanowires and nanowires of oxides and other compounds. At T =90%, R s values for CNTs are 60–400 Ω sq −1 , for metal nanowires 10–30 Ω sq −1 , for TiN nanofibres 100–200 Ω sq −1 and for oxide nanowires 2,000–10,000 Ω sq −1 (refs 1 , 15 , 17 , 21 , 31 , 32 , 33 , 34 ). Metal nanowire TCEs have shown great promise in reaching excellent performance because of the high conductivity of metals. Various methods have been used to improve performance, including increasing the nanowire length to increase transport distance [21] , [32] , decreasing the diameter to reduce the light scattering and annealing of nanowire junction to reduce resistance by thermo, electrochemical or nanoplasmonic welding [14] , [31] , [35] . The best performance of metal nanowire TCEs has reached R s =10 Ω sq −1 at T =90% (ref. 32 ). A fundamental question is how to improve the R s –T performance of metal nanowire TCEs with a large leap. This is important, as it can reduce the power loss in many optoelectronic devices. Here we introduce a mesoscale metal-wire concept in conjunction with metal nanowire networks to realize an order of magnitude reduction in sheet resistance at a given transmittance. Through computer simulation, we first predict the extraordinary R s –T performance enhancement of mesoscale metal wires. Then, this mesoscale metal-wire concept is realized by lithography, in which we demonstrate the metal-wire network TCE having a performance as high as 0.36 Ω sq −1 of sheet resistance and 92% of transmittance. Electrochromic devices exhibit a significantly improved colour-switching time by applying the mesoscale metal wires. These results prove the applicability of the mesoscale metal wires and their advantages in enhancing energy efficiencies of modern optoelectronic devices. Mesoscale metal wires The fundamental concept of using mesoscale metal wires is illustrated in Fig. 1a , where the mesoscale wires have widths from 1 to 5 μm. We call these metal-wires mesoscale, as their widths and spacings are between two types of electrical connections in nanowire TCE optoelectronic devices: metal nanowires and macroscopic metal lines. First, mesoscale wires are one order of magnitude larger than metal nanowires (50–300 nm), although they are one order of magnitude smaller than macroscopic metal lines (~50 μm) that are typically made by screening printing in solar cell devices. Second, the spacing of mesoscale wires here is around several 100 μm, whereas the spacing of nanowires is several 100 nm to a few μm and the spacing of macroscopic wires is several mm. The spacing for certain width of metal wires is generally kept above certain values in order to maintain adequate optical transmittance based on different applications. When combining mesoscale wires with nanowires and macroscopic wires, we can promote the electron conduction over multiple length scale with minimum power loss. Here nanowire networks no longer need to transport electrons to a several millimetre long distance as in the combination of only nanowires and macroscopic metal wires. Nanowires here only need to transport electrons several 100 μm distance, whereas the transport of electrons across several millimetre distance is carried out by mesoscale wires with much higher conductance. 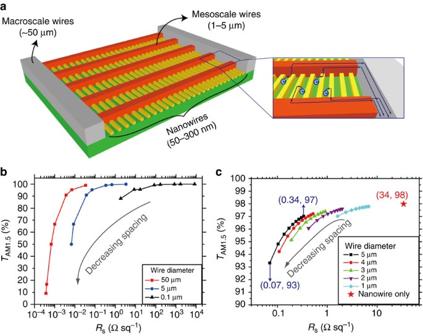Figure 1: Mesoscale metal-wire network TCE concept. (a) Schematic of mesoscale design (not drawn to scale). The mesoscale metal-wire network between the nanowire transparent electrode and macroscale wires (metal fingers) can shorten the carrier transport distance and enhance theRs–Tperformance. (b) SimulatedRs–Tcurves of metal wires with various diameters. The wire spacings are 5, 10, 50, 100, 500, 1,000 and 5,000 μm. For 100-nm nanowires, spacing of 1 μm is also included. (c) SimulatedRs–Tperformance of metal-wire transparent electrode with the mesoscale metal microwire layer. The diameter and spacing of metal nanowires are 50 nm and 5 μm, respectively. The spacings of metal mesoscale wires are 100, 150, 200, 250, 300, 350, 400, 450 and 500 μm. Figure 1: Mesoscale metal-wire network TCE concept. ( a ) Schematic of mesoscale design (not drawn to scale). The mesoscale metal-wire network between the nanowire transparent electrode and macroscale wires (metal fingers) can shorten the carrier transport distance and enhance the R s – T performance. ( b ) Simulated R s – T curves of metal wires with various diameters. The wire spacings are 5, 10, 50, 100, 500, 1,000 and 5,000 μm. For 100-nm nanowires, spacing of 1 μm is also included. ( c ) Simulated R s – T performance of metal-wire transparent electrode with the mesoscale metal microwire layer. The diameter and spacing of metal nanowires are 50 nm and 5 μm, respectively. The spacings of metal mesoscale wires are 100, 150, 200, 250, 300, 350, 400, 450 and 500 μm. Full size image R s –T simulation The important benefits of introducing mesoscale wires into nanowires and macroscopic wires to form multiscale networks can be understood from the R s –T performance simulation. Figure 1b shows the simulation results when using only single scale of parallel wire arrays. Here we use square cross-section wires for simplicity to demonstrate the trend. The diameters are 100 nm for nanowires, 5 μm for mesoscale wires and 50 μm for macroscopic wires, respectively. The data points on each curve represent different wire spacings, which are 5, 10, 50, 100, 500, 1,000 and 5,000 μm. For 100-nm nanowires, spacing of 1 μm is also included to better manifest the curve trend. For the optical transmittance, geometrical optics is used for mesoscale and macroscale wires, as their diameters and spacings are much larger than the wavelength, and rigorous coupled-wave analysis is used for nanowires. For sheet resistance simulation, a typical bulk resistivity of metal is used (see Methods). There is interesting observation from this simulation. When the spacings between wires are large enough, all three scales of wires alone can have high T >95%. The spacings need to be >1,000 μm for macroscale, >100 μm for mesoscale and >5 μm for nanoscale wires, respectively. However, R s at T >95% falls in completely different regimes for these three scales of wires: 10 −3 –10 −1 Ω sq −1 for macroscale, 10 −2 –10 1 Ω sq −1 for mesoscale, 10 1 –10 4 Ω sq −1 for nanoscale, respectively. From only the R s –T performance standpoint, the macroscale wires are better than the smaller ones, as R s has quadratic dependence on diameter, whereas T only has linear dependence in the regime of diameter and spacing much larger than wavelength of the light. However, transporting electrons to or from local areas in optoelectronic devices needs small diameter wires (nanowires), as the spacings in macroscale wires are too large to carry out this function and will cause huge ohmic loss. On the other hand, from the spacing and sheet resistance shown above, nanoscale wires alone have inferior R s – T performance and thus are not efficient enough to transport electrons to or from macroscale wires. The integration of mesoscale wires and nanowires combines both advantages: great R s – T performance and local conductance. This will effectively reduce the power loss even at high transmittance regime. Figure 1c shows such a large improvement of nanowire arrays by incorporating mesoscale wires. Here we choose the dimension of parallel nanowire array transparent electrode to be 50 nm in wire diameter and 5 μm in wire spacing and calculated its ( R s , T )=(34 Ω sq −1 , 98%) and applied the parallel mesoscale metal-wire arrays with different diameters (1, 2, 3, 4 and 5 μm) to form a two-scale hybrid metal-wire transparent electrode. The spacings of mesoscale wires are varied from 100 to 500 μm (see Figure caption). The result proves the effectiveness of the mesoscale metal-wire network. For instance, when the mesoscale wire array with 5 μm in diameter is 500 and 100 μm in spacing, the R s – T performance is enhanced from (34 Ω sq −1 , 98%) for nanowire alone to (0.34 Ω sq −1 , 97%) and (0.07 Ω sq −1 , 93%) for hybrid wires, respectively, which is 100–1,000 times more conducting but only has little drop in T . This high level of R s – T performance has not been seen in any previous studies. Metal mesowires incorporated with nanowire TCEs To experimentally demonstrate the importance of mesoscale wire concept, e-beam lithography was employed to fabricate the gold nanowire (AuNW) array on quartz wafers, followed by copper mesoscale wire (CuMW) array made by photolithography with the direction perpendicular to the nanowire, as shown in Fig. 2a . The fabricated wires have rectangular shapes. The dimensions of AuNWs are 270 nm in width ( Supplementary Fig. S1 ), 120 nm in height and 5 μm in spacing, and those of CuMWs are 5 μm in width, 2.8 μm in thickness with spacing ranging from 200 to 500 μm. (details in Figure caption). As shown in Fig. 2b , the R s – T performance of AuNWs array alone was measured to be R s =7.2 Ω sq −1 and T =95%, consistent with optical simulation, whereas the hybrid of AuNWs and CuMWs can achieve 0.36 Ω sq −1 at T =92%, showing an order of magnitude improvement in R s with little change in T . This result shows that the mesoscale design can greatly exceed the traditional limit of single-layer transparent electrodes. 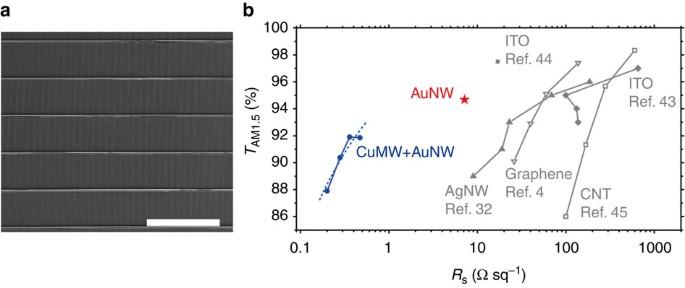Figure 2: Meso- and nano-scale metal-wire network TCEs. (a) SEM images of the metal-wire network consisting of AuNWs and CuMWs. The scale bar is 400 μm. (b) MeasuredRs–Tperformance of nanowire arrays and mesoscale metal-wire network transparent electrode. The dimensions of AuNWs are 270 nm in width, 120 nm in height and 5 μm in spacing, and CuMWs are 5 μm in width, 2.8 μm in thickness with 200, 300, 400 and 500 μm in spacing. The CuMW mesoscale layer greatly reduces the sheet resistance of AuNW arrays. Other types of transparent electrodes, including AgNWs32, ITO43,44, graphene4and CNTs45were also included for comparison. Figure 2: Meso- and nano-scale metal-wire network TCEs. ( a ) SEM images of the metal-wire network consisting of AuNWs and CuMWs. The scale bar is 400 μm. ( b ) Measured R s – T performance of nanowire arrays and mesoscale metal-wire network transparent electrode. The dimensions of AuNWs are 270 nm in width, 120 nm in height and 5 μm in spacing, and CuMWs are 5 μm in width, 2.8 μm in thickness with 200, 300, 400 and 500 μm in spacing. The CuMW mesoscale layer greatly reduces the sheet resistance of AuNW arrays. Other types of transparent electrodes, including AgNWs [32] , ITO [43] , [44] , graphene [4] and CNTs [45] were also included for comparison. Full size image We note that microscale metal wire array transparent electrodes have been reported previously [36] , [37] . However, the R s – T enhancement was not as prominent as our work. The key difference lies in the thickness of the mesowires. As increasing thickness does not significantly affect the transmittance, for highly conducting mesowire, the thickness must be comparable to the width; therefore, the sheet resistance can be reduced without sacrificing transmittance. Electrospun metal mesowires For a more facile, lithography-free demonstration of our mesoscale metal network design, we developed the electrospinning process to produce ultra-long copper mesoscale wires with ~1 μm in diameter, which were used in conjunction with Ag nanowire networks developed previously by our group and others [2] , [14] , [31] , [32] , [38] . Electrospinning is a powerful technique to produce polymer wires with diameters ranging from sub-100 nm to few micrometres. In the past decade, it has been also used to produce wires of a variety of inorganic materials [39] . Our group has previously used electrospinning for making Cu nanowires for transparent electrodes [15] , [16] . Here we extend this method for making larger diameter mesoscale wires. The process flow is illustrated in Fig. 3 . First, a grounded metal piece was used as a wire collector, and the electrical field formed by the two edges in the middle can align the electrospun polymer nanowires across the 1-inch wide gap [40] . Then, 1 μm of copper was deposited on the nanowires using thermal evaporation to form the free-standing and aligned CuMWs. The wire density and thus the spacing can be easily controlled by electrospinning time period. This is particularly advantageous comparing with expensive photolithography process. In the transfer step, alcohol was applied to the silver nanowire (AgNW) substrate to dissolve the polymer core away and also generate capillary force to pull the CuMWs towards the substrate during solvent evaporation. The transfer step is followed by a roll-pressing process to further ensure the contact between intersecting wires. The subsequent annealing fuses both AgNW–AgNW junctions and AgNW–CuMW junctions, thereby creating a continuous conducting pathway. The aligned configuration of AgNW–CuMW transparent electrodes is characterized using a scanning electron microscope (SEM), as shown in Fig. 4a . For the demonstration of the fused junction between CuMW and AgNWs, a sacrificial polymer film was used for the subsequent lift-off the AgNW–CuMW network; therefore, we could characterize the morphology from the back side. As shown in Fig. 4b , the CuMW and the intersecting AgNW are fused into each other, guaranteeing low contact resistance between the nanoscale layer and the mesoscale layer. Additional SEM images are included in Supplementary Fig. S2 . The electrospun free-standing CuMWs can also be applied to other types of transparent electrodes. This great versatility makes our mesoscale concept applicable to various kinds of optoelectronic devices with special requirement for transparent electrode—for example, conduction/valence band position, buffer layer and so on. Here we transferred the CuMWs on not only AgNW network but also ITO, AZO, poly(3,4-ethylenedioxythiophene):poly(styrenesulfonate) (PEDOT:PSS), and bare glass substrates and compared their R s – T performances ( Fig. 4c ). The result shows great effectiveness of CuMWs in improving the R s – T performances of various transparent electrodes. The ( R s , T ) of only CuMW lie in the range of 0.15 Ω sq −1 , 85% to 0.64 Ω sq −1 , 97%, depending on the wire density controlled by electrospinning time. After incorporating conventional TCEs with CuMWs, all sheet resistances of the sample were improved to below 0.4 Ω sq −1 , with <3% change in transmittance. Based on the shift of ( R s , T ) value, the average ( R s , T ) of electrospun CuMWs can be calculated to be (0.40±0.05 Ω sq −1 , 97.1±0.6%), which again demonstrates the outstanding R s – T performance of mesoscale metal-wire networks. Cross-array of CuMWs can also be made by performing the transfer process twice in orthogonal directions, as shown in Supplementary Fig. S3 . As the underlying TCE and CuMWs are in parallel configuration, the resulting sheet resistance is shifted closer to the values of CuMWs, and the transmittance is the product of TCE and CuMWs. These promising results prove that our mesoscale metal-wire network concept is compatible with traditional TCEs. Using electrospun free-standing CuMWs as a facile yet effective approach, the power loss of TCEs can be significantly decreased. 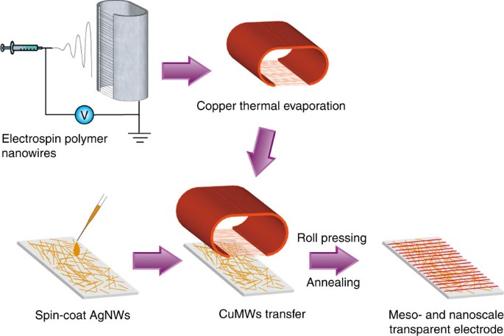Figure 3: Incorporation of metal mesowires using electrospinning. First, the polymer nanowires are electrospun and aligned on the grounded collector. The collector has two parallel edges that are 1 inch apart. Copper thermal evaporation was employed on the polymer nanowires up to 1 μm thickness. These free-standing CuMWs were then transferred onto an as-made AgNW transparent electrode, followed by roll pressing and Ar annealing for junction fusion. Figure 3: Incorporation of metal mesowires using electrospinning. First, the polymer nanowires are electrospun and aligned on the grounded collector. The collector has two parallel edges that are 1 inch apart. Copper thermal evaporation was employed on the polymer nanowires up to 1 μm thickness. These free-standing CuMWs were then transferred onto an as-made AgNW transparent electrode, followed by roll pressing and Ar annealing for junction fusion. 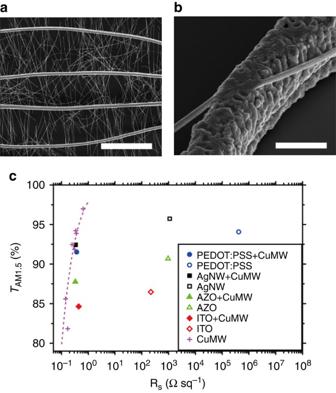Figure 4:Rs–Tperformance enhancement of different kinds of TCEs. (a) SEM image of the aligned CuMWs and the underlying AgNWs. The scale bar is 20 μm. (b) High-magnification tilted view of the CuMW/AgNW-fused junction. The scale bar is 1 μm. Note that, in order to observe the junction locating below CuMWs, the metal-wire network was lifted off from the original substrate and flipped to the back side. (c)Rs–Tperformance of electrospun CuMWs and the improvement of various kinds of transparent electrodes. All transparent electrodes are significantly improved after adding the mesoscale metal-wire layer. Their sheet resistances decrease to <0.4 Ω sq−1with only <3% of transmittance change. Full size image Figure 4: R s – T performance enhancement of different kinds of TCEs. ( a ) SEM image of the aligned CuMWs and the underlying AgNWs. The scale bar is 20 μm. ( b ) High-magnification tilted view of the CuMW/AgNW-fused junction. The scale bar is 1 μm. Note that, in order to observe the junction locating below CuMWs, the metal-wire network was lifted off from the original substrate and flipped to the back side. ( c ) R s – T performance of electrospun CuMWs and the improvement of various kinds of transparent electrodes. All transparent electrodes are significantly improved after adding the mesoscale metal-wire layer. Their sheet resistances decrease to <0.4 Ω sq −1 with only <3% of transmittance change. Full size image Electrochromic device demonstration PEDOT-based electrochromic devices were assembled to demonstrate the effectiveness of our mesowires in terms of coloration response time. For PEDOT, the colour is light blue when at +0.2 V and dark blue when at −0.4 V. The cyclic voltammetry diagram and the redox peak positions can be found in other literature [41] . Here the potential of the PEDOT electrochromic device is switched between +0.2 and −0.4 V. The potential switches instantaneously; however, it takes time to complete the colour-state transition because of the kinetics of doping and undoping process inside the electrochromic material. In Fig. 5 , we measure the transmittance response to the potential cycles. The result clearly shows a much shorter colour-switching time using CuMW/ITO as the transparent electrode comparing to only ITO. Take bleaching for example; the switching time (Δ t bleach ) to reach 90% of colour-state change for ITO is 12.2 s; however, CuMW/ITO only takes 3.1 s, which is four times faster. Although the potential steps are the same, lower ohmic resistance of the transparent conducting substrate results in higher current, and thus the colouration and bleaching processes proceed faster with the CuMW/ITO transparent electrode. Moreover, lower sheet resistance means less power dissipation and higher energy efficiency. As electrochromic devices are generally used as large-area smart windows, the change of colour-switching time and power dissipation because of different R s – T performance will be even more significant. A side-by-side comparison video can be found in Supplementary Movie S1 . This electrochromic device demonstration again serves as a strong evidence of the advantage of metal mesowires. 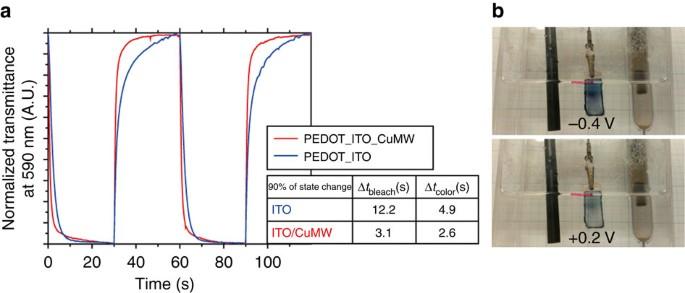Figure 5: Electrochromic device demonstration. (a) Normalized PEDOT:PSS electrochromic device transmittance response versus time. The potential of PEDOT is switched between +0.2 V (bleached) and −0.4 V (colour) versus Ag/AgCl, and the duration is 30 s. The colour-switching time of ITO/CuMW transparent electrode is much faster than ITO. (b) The photo of the experimental setup and comparison between the colour state (−0.4 V) and the bleach state (+0.2 V). The components from left to right are: the graphite counter electrode, the PEDOT:PSS electrochromic thin film and the Ag/AgCl reference electrode. The electrolyte is 1 M LiClO4in acetonitrile. The size of electrochromic sample is 1 × 2.54 cm2. Figure 5: Electrochromic device demonstration. ( a ) Normalized PEDOT:PSS electrochromic device transmittance response versus time. The potential of PEDOT is switched between +0.2 V (bleached) and −0.4 V (colour) versus Ag/AgCl, and the duration is 30 s. The colour-switching time of ITO/CuMW transparent electrode is much faster than ITO. ( b ) The photo of the experimental setup and comparison between the colour state (−0.4 V) and the bleach state (+0.2 V). The components from left to right are: the graphite counter electrode, the PEDOT:PSS electrochromic thin film and the Ag/AgCl reference electrode. The electrolyte is 1 M LiClO 4 in acetonitrile. The size of electrochromic sample is 1 × 2.54 cm 2 . Full size image Through simulation and experiments, we have shown the powerful concept of mesoscale metal wire to decrease the sheet resistance of nanowire TCE by orders of magnitude with only little compromise on optical transmittance. The mesoscale metal wires that are several micrometres in diameter provide large cross-section area for electron transport, thereby enhancing the R s – T performance. By the incorporation of mesoscale metal wires, various types of TCEs show great improvement in the performance, such as AgNWs, ITO and PEDOT:PSS. The carriers first transport within the underlying TCE only for several 100 μm and then they are collected and transported into the highly conducting mesowires; therefore, the ohmic loss can be greatly mitigated. In electrochromic devices, lower ohmic loss leads to higher current and faster colour-switching speed, which are desirable in practical application. This mesoscale metal-wire design can be also materialized by the electrospinning technique without using shadow masks or lithography. We believe the outstanding performance and the wide applicability of our mesoscale metal-wire concept can provide great opportunities for the optoelectronic devices to become more energy efficient. R s – T simulation For simplicity, we let the cross-section of metal wires to be square-shaped with side length a . For 100-nm wire arrays, the optical transmittance simulation was performed using rigorous coupled-wave analysis. The transmittance spectra (400–1,100 nm) were then weighed for AM1.5 solar spectrum to derive the average transmittance, T AM1.5 . For wire arrays larger than 1 μm, the optical transmittance was calculated by geometrical shadow loss—that is, T=S/(S+a) × 100%, where S is the wire spacing. For sheet resistance simulation, with the assumption of constant electrical conductivity, we can derive R s =ρ ( S+a )/ a 2 , where ρ =16.8 Ω nm. Lithographically fabricated metal-wire network The nanowire arrays were fabricated on quartz wafers by standard e-beam lithography using MMA/PMMA (MicroChem) as e-beam resist, followed by thermal evaporation of chromium/gold (7 nm/120 nm) and lift-off process in acetone. The size of array is 5 × 5 mm 2 . The mesoscale wire arrays were fabricated on the same sample by photolithography using 7-μm SPR220 photoresist. The orientation was orthogonal to the gold nanowire arrays previously made by e-beam lithography. Chromium/copper (7 nm/2.8 μm) was then thermally evaporated, followed by lift-off process in acetone. Electrospun-evaporated metal mesowires Fourteen wt % of polyvinylpyrrolidone (PVP, MW=1.3 × 10 6 g mol −1 , Acros) and anhydrous ethanol (Sigma-Aldrich, 99.5%) solutions were made for electrospinning. The solution was loaded in a syringe with a needle tip, which is connected to a voltage supply (ES30P-5W, Gamma High Voltage Research). The applied potential on the needle was +4 kV. The distance between the syringe needle tip and the grounded collector was 15 cm, and the pump rate was 0.15 ml h −1 . High electrical potential and surface charges pulled polymer nanowires out of the droplet in front of the needle, and the nanowires were attracted towards the collector, forming free-standing nanowires lying across two edges of the collector. Different electrospinning time can be chosen for desired nanowire densities. Thermal evaporator (M. Braun) was then used for Cu deposition on electrospun nanowires. Seven nanometre of Cr (Kurt J. Lesker) was deposited on electrospun nanowires first for better adhesion and then 1 μm of Cu (99.99%, Kurt J. Lesker) was deposited. Several drops of ethanol were put on the surface of as-made transparent electrodes before the CuMWs were transferred to them. A calender machine (MTI Corp.) was used to ensure better physical contacts between CuMWs and the transparent electrode. Post annealing at 200 °C for 40 min in Ar atmosphere was employed for junction fusion. AgNW transparent electrodes The synthesis method of AgNWs can be found in other papers [42] . A mixture of 0.334 g PVP and 20 ml ethylene glycol (Sigma-Aldrich) was heated at 170 °C in a three-neck glass flask, and then 0.025 g of silver chloride (Sigma-Aldrich) was finely ground and added to the flask for initial nucleation of the silver seeds. After 3 min, 0.110 g of silver nitrate (Sigma-Aldrich), the actual silver source, was titrated for 10 min, followed by an additional 30 min of heating for completing the reaction. The solution was then cooled down and centrifuged three times at 6,000 r.p.m. for 30 min to remove ethylene glycol, PVP and other impurities in the supernatant. After the final centrifugation, the precipitates of AgNWs were redispersed in 30 ml of methanol. The transparent electrodes were made by spin coating (WS-400-6NPP, Laurell) the AgNW dispersion, and their transmittance and sheet resistance were tuned by concentrations, rotational speed and spin-coating times. AZO transparent electrodes The AZO layers were deposited by atomic layer deposition [16] (Savannah, Cambridge NanoTech) with trimethylaluminium (97%, Sigma-Aldrich) and diethylzinc (DEZ, Zn 52.0 wt %, Sigma-Aldrich) as precursors. The deposition temperature was 150 °C, and the idle pressure was 0.5 Torr. One cycle of ZnO or Al 2 O 3 was made by 15 ms pulse of water followed by 15 ms pulse of DEZ or trimethylaluminium, and the chamber was allowed to pump for 20 s to remove excess precursors. One supercycle of AZO is achieved by 25 ZnO cycles and one Al 2 O 3 cycle. The transmittance and sheet resistance were controlled by different numbers of supercycle. ITO transparent electrodes The ITO thin film was coated by sputtering technique (ATC Orion, AJA International Inc.). The commercial ITO target was sputtered using 125 watts of RF power under 2.5 m Torr of Ar/O 2 environment for different periods of time to synthesize ITO thin film with different sheet resistance. The flow rates of Ar and O 2 were 19 and 1 sccm, respectively. PEDOT:PSS transparent electrodes The PEDOT:PSS (1.3 wt % aqueous solution, Sigma-Aldrich) was bought from Sigma-Aldrich. The transparent electrodes were made by spin coating PEDOT:PSS solution on glass slides at 4,000 r.p.m. for 30 s. The transmittance and sheet resistance were controlled by different times of spin coating. Electrical and optical property measurement The transmittance measurement used a quartz tungsten halogen lamp as the light source, coupled with a monochromator (Newport 70528) to control the wavelength. An iris and a convex lens were used to focus the beam size to about 1 mm × 2 mm, and a beam splitter split the light beam into an integrating sphere (Newport) for transmittance measurement and a photodiode (Newport, 818-UV-L). The photodiode is connected to an electrometer (Keithley 6517A) for light intensity calibration. The samples were placed in front of the integrating sphere; therefore, both specular transmittance and diffuse transmittance were included. An identical glass slide was used for reference. A source-measure unit (Keithley 236) was used to measure the photocurrent from the integrating sphere, and the transmittance spectrum was thus calculated based on the reference plain glass slide. The transmittance spectrum was then weighed by solar spectrum from 400 to 800 nm to obtain the average transmittance T AM1.5 . For the sheet resistance measurement, two contacts were drawn by a silver pen (CircuitWorks, ITW Chemtronics), separated by a square area of transparent electrode, and then the resistance was measure by a zero-calibrated multimeter. A comparison between two-probe- and four-probe resistance measurements can be found in Supplementary Table S1 . The differences of the resistance values measured by these two methods are very small. The R s – T curves in Fig. 2b (blue dash curve) and Fig. 4c (purple dash curve) are fitted based on percolation theory. The fitting parameters and method are detailed in Supplementary Fig. S4 . Characterization All the SEM images were taken by an FEI Nova NanoSEM. For the observation of CuMW–AgNW junction, PMMA sacrificial layer was first spin-coated on a glass slide, followed by the normal CuMW–AgNW fabrication process mentioned previously. The sample was then immersed in acetone to dissolve the PMMA sacrificial layer and transferred on a silicon wafer with AgNW side on top. Electrochromic device demonstration The electrochromic samples were made by drop casting 0.13% of PEDOT:PSS aqueous solution (Sigma-Aldrich) on transparent electrodes with the size of 1 × 2.54 cm 2 . The CuMWs were transferred on glass slides and sputtered with 100 nm of ITO, followed by 20 nm of atomic-layer-deposited AZO for passivating CuMWs. Bared glasses coated with the same thickness of ITO and AZO were also coated with PEDOT for comparison. A standard three-electrode setup (BioLogic) was employed on the electrochromic sample to manipulate the potential, with a graphite rod as the counter electrode and Ag/AgCl as the reference electrode (Accumet). The electrolyte was 1 M LiClO 4 (Alfa Aesar) in acetonitrile (EMD Chemicals). The electrochromic electrode was applied with the potential steps of +0.2 and −0.4 V for colour changing for 30 s. In the meantime, the transmittance at 590 nm was measured and recorded using a spectrophotometer (Shimadzu, UV-1700). How to cite this article: Hsu, P.-C. et al. Performance enhancement of metal nanowire transparent conducting electrodes by mesoscale metal wires. Nat. Commun. 4:2522 doi: 10.1038/ncomms3522 (2013).